GATA simple sequence repeats function as enhancer blocker boundaries Simple sequence repeats (SSRs) account for ~3% of the human genome, but their functional significance still remains unclear. One of the prominent SSRs the GATA tetranucleotide repeat has preferentially accumulated in complex organisms. GATA repeats are particularly enriched on the human Y chromosome, and their non-random distribution and exclusive association with genes expressed during early development indicate their role in coordinated gene regulation. Here we show that GATA repeats have enhancer blocker activity in Drosophila and human cells. This enhancer blocker activity is seen in transgenic as well as native context of the enhancers at various developmental stages. These findings ascribe functional significance to SSRs and offer an explanation as to why SSRs, especially GATA, may have accumulated in complex organisms. Genome sequence analysis has revealed the presence of a large proportion of non-coding DNA in complex organisms. Much of this non-coding DNA consists of a variety of repetitive DNA including transposable elements (TEs) and simple sequence repeats (SSRs). Certain repetitive sequences have been implicated in chromatin-mediated transcriptional regulation, chromosome organization, imprinting, chromatin domain boundary function and complex nuclear features such as heterochromatin, telomeres and nucleolar organization [1] , [2] , [3] , [4] , [5] , [6] , [7] , [8] . SSRs, on the other hand, have not been directly implicated in such regulatory roles although this class of DNA has also accumulated in complex genomes, particularly in vertebrates [9] , [10] . We have reported earlier that only selected SSRs have been favoured [9] and one of the most prominent of those SSRs is the GATA repeat. GATA repeat elements (GEs), which are highly abundant on the sex chromosomes of several organisms, have GATA 10–12 as the most abundant size of this repeat and are present almost exclusively in the intergenic regions [10] . GATA repeats have also been found to be associated with genes that are expressed early during development while the GE-devoid region of Y chromosome contains genes that are expressed late during spermatogenesis. We also noticed a frequent association of matrix attachment region (MAR) potential sequences with the GATA repeats [10] . MAR DNA, by its association to the nuclear matrix, creates chromatin domains that are topologically constrained, which helps in regulating genes and organizing the genome in eukaryotes [11] , [12] , [13] , [14] , [15] . These observations suggested a gene regulation and genome packaging-related function for this SSR element. Here, we show that GATA repeats function as enhancer blocker in human cells and Drosophila . These findings bring to light the regulatory role of SSRs and may explain why complex genomes have accumulated such repetitive elements. GATA SSR functions as enhancer blocker in human cells To test our hypothesis that GATA has gene regulatory function, GATA-rich regions from the human Y chromosome ( Supplementary Fig. S1 ) were taken and tested for enhancer blocker function using colony formation assay in K562 human cell line. The test fragments were placed between the mHS2 enhancer and γ-globin promoter-driven neomycin resistance gene ( neo R ) to test if they block the access of the enhancer to the promoter ( Fig. 1a ). If a sequence acts as a boundary or enhancer blocker, it would prevent mHS2 to talk to neo R , resulting in its lower expression and thus low numbers of resistant colonies. A known boundary element, cHS4 enhancer blocker from β-globin locus [16] , was used as a positive control in the assay. To have comparable results, equal numbers of cells were transfected with same amounts of the various DNA constructs. We observed that all the GATA-containing fragments show enhancer blocker activity with the two GEs from human Y chromosome, GE7 (389 bp) and GE10 (930 bp), showing boundary activity comparable to that of cHS4 ( Fig. 1a ). 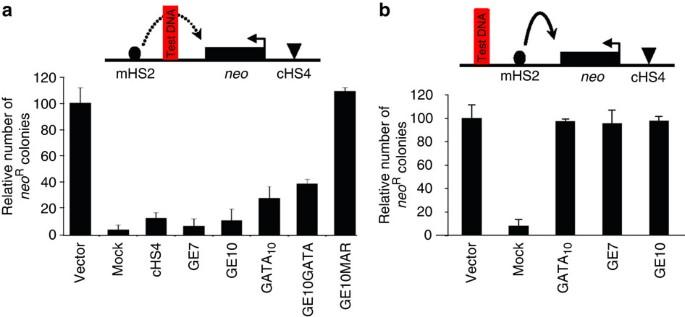Figure 1: GATA repeat has enhancer blocker activity in human K562 cells. (a) A cartoon representing the enhancer blocker assay construct that carries aγ-globin/neomycin(neo) gene driven by mHS2 enhancer from LCR of chickenβ-globinlocus (upper panel). The graph shows relative number of neomycin-resistant colonies in the presence of the corresponding constructs as compared with that in the case of transfection with vector DNA. The error bars represent s.d. from mean. Vector alone and mock, that is, without any DNA serve as positive and negative controls forneosensitivity, respectively. Construct has chickenβ-globinblocker, cHS4, as positive control for enhancer blocker activity, while GE7, GE10, GATA10, GE10-GATA and GE10-MAR were the test fragments. (b) A bar graph of the relative neomycin-resistant colonies in corresponding constructs with respect to vector alone when the GE is placed upstream to the enhancer. Similar number of neomycin-resistant colonies in all constructs as compared with vector shows that GE is not a repressor. Figure 1: GATA repeat has enhancer blocker activity in human K562 cells. ( a ) A cartoon representing the enhancer blocker assay construct that carries a γ - globin / neomycin ( neo ) gene driven by mHS2 enhancer from LCR of chicken β - globin locus (upper panel). The graph shows relative number of neomycin-resistant colonies in the presence of the corresponding constructs as compared with that in the case of transfection with vector DNA. The error bars represent s.d. from mean. Vector alone and mock, that is, without any DNA serve as positive and negative controls for neo sensitivity, respectively. Construct has chicken β-globin blocker, cHS4, as positive control for enhancer blocker activity, while GE7, GE10, GATA 10 , GE10-GATA and GE10-MAR were the test fragments. ( b ) A bar graph of the relative neomycin-resistant colonies in corresponding constructs with respect to vector alone when the GE is placed upstream to the enhancer. Similar number of neomycin-resistant colonies in all constructs as compared with vector shows that GE is not a repressor. Full size image The GE sequences used in the boundary assay, along with 20-kb additional flanking region both at 5′ and 3′ end, were tested for MAR potential using MAR-Wiz finder [17] ( Supplementary Fig. S1 ). Although the MAR region coincided with GATA repeat only in GE10, both GE7 and GE10 showed comparable boundary activity. Thus, we decided to test whether GATA repeat or MAR or both contribute to the boundary function assayed here. We used the GATA-rich region (GE10GATA, 160 bp) and the GATA-devoid or MAR region of GE10 (GE10MAR, 727 bp) separately as test fragments for this purpose. The results show that the boundary activity of GE10 is confined to the GATA-rich region and that MAR region has no boundary function ( Fig. 1a ). To further confirm whether the boundary activity is solely due to the GATA tetranucleotide repeats, a synthetic GATA 10 sequence (40 bp) was also used as a test fragment in this assay ( Fig. 1a ). We observed enhancer blocker activity with synthetic GATA repeat itself. All these results together indicate that GATA SSR can act as an enhancer blocker boundary in human cell line. GATA repeats function as enhancer blocker in Drosophila Boundary elements are known to function across species [16] , [18] , [19] and Drosophila melanogaster is used as a model system of choice to study such elements from different species taking genetic and cell biology approaches in the transgenic context [20] , [21] , [22] . Before going for transgenic experiments, we checked whether GATA repeats bind to specific proteins in the Drosophila embryo nuclear extract. Gel-shifts using GATA 3 , GATA 8 and GATA 11 as probes, clearly indicated that GATA 11 has the ability to bind proteins more efficiently than GATA 3 and GATA 8 ( Supplementary Fig. S2a ). We also saw that the DNA–protein complex with longer repeat GATA 11 cannot be competed efficiently by shorter repeats ( Supplementary Fig. S2b ), suggesting that GATA-interacting protein prefers longer GATA repeats. These results indicate towards the presence of the GATA SSR function in fly and that fly can be used as a model to study it. We use a transgene-based enhancer blocker assay where test fragments are placed between fushi-tarazu (ftz) enhancer and hsp70 promoter-driven lacZ gene ( Fig. 2a ) [23] . GE5 (394 bp), GE7 (389 bp) and GE10 (930 bp) from the human Y chromosome ( Supplementary Fig. S1 ) were tested for boundary activity in this assay. We compared our results with the ‘vector’ control line containing no test DNA and blocker control line of ‘ Su(Hw) 5 ’ (355 bp) as test fragment [23] . Genetic tools available in Drosophila enabled us to flip-out the test fragments from the transgenes using Cre recombinase-expressing fly and compare reporter activity in presence and absence of the test fragment while keeping the genomic context unchanged ( Fig. 2a ) [24] . A significant increase in the LacZ staining for flipped-out lines as compared with initial lines is seen, establishing that the decrease in LacZ staining in the boundary lines is exclusively due to the presence of GE between the ftz enhancer and the lacZ gene ( Fig. 2b ). The quantification of staining by ImageJ—an image analysis software—shows similar results too ( Supplementary Fig. S3a ). We also checked the enhancer blocker activity of only GATA and only MAR parts of GE10 as done in the human cell line. We found no significant change in the LacZ staining intensity in the initial versus the flipped-out MAR line ( Supplementary Fig. S3b ), indicating that MAR does not function as boundary. When synthetic GATA 10 (40 bp) was used as the test fragment in the assay, reduction in LacZ staining was clearly seen ( Fig. 2b , Supplementary Fig. S3a ), confirming that GATA by itself is sufficient for the boundary activity. It should also be noted that the enhancer blocker activity is not a property of any repetitive element but rather is an attribute of GATA SSR exclusively, as earlier reports from our lab have shown that GAGAG repeat fails to act as a boundary despite GAGAG motif having the ability to recruit GAGA boundary factor [25] . 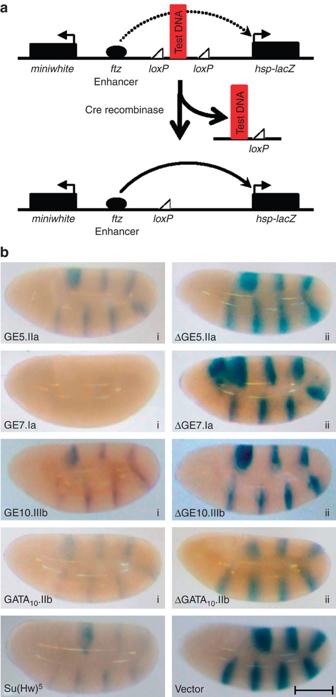Figure 2: Enhancer blocker activity of GATA inDrosophila. (a) The enhancer blocker assay construct, CfhL vector, that carriesminiwhitegene as transformation marker andhsp70promoter-drivenlacZwithftzseven-stripe enhancer as the reporter.loxPsites are shown as triangles. (b) LacZ staining of embryos. While the initial lines (i) containing the boundary element (shown as red bar) block the enhancer–promoter communication, seen as weaklacZexpression, flipped-out lines (ii) lose this ability, seen as significantly stronger staining in corresponding lines. Su(Hw)5and vector serve as positive and negative controls, respectively. The scale bar drawn on bottom right of the panel measures 100 μm in length. Figure 2: Enhancer blocker activity of GATA in Drosophila . ( a ) The enhancer blocker assay construct, CfhL vector, that carries miniwhite gene as transformation marker and hsp70 promoter-driven lacZ with ftz seven-stripe enhancer as the reporter. loxP sites are shown as triangles. ( b ) LacZ staining of embryos. While the initial lines (i) containing the boundary element (shown as red bar) block the enhancer–promoter communication, seen as weak lacZ expression, flipped-out lines (ii) lose this ability, seen as significantly stronger staining in corresponding lines. Su(Hw) 5 and vector serve as positive and negative controls, respectively. The scale bar drawn on bottom right of the panel measures 100 μm in length. Full size image GATA functions as boundary and not as repressive element In our assay systems, the reduction in the reporter gene activity in the enhancer blocker assays can also be explained by alternative mechanism if the test fragment were to function as repressor. To rule out the repressor function of GE, we checked the effect of GATA/GEs when placed upstream of the enhancer in human cells. Unlike in enhancer blocker constructs where GEs and GATA 10 block enhancer–promoter interaction, when placed upstream to the mHS2 enhancer, they have no effect on the neomycin resistance gene expression. This rules out any repressor effect associated with GATA ( Fig. 1b ). In our experiments in the fly system, the reduction of LacZ staining, on which the assay is based, could have also been due to either genomic position of the transgene or a repressive property of the test element. First, to rule out the possibility of any genomic position effect, several independent lines of each construct were tested for their boundary activity and their average boundary strength was quantitated using Image J software ( Supplementary Table S1 ). Our results show that irrespective of the genomic context, every time the GE fragment is flipped out there is an enhancement in the lacZ expression, indicating that the initial low lacZ expression is due to the boundary effect of the GE. Thus, the flip-out experiment separates out the position effect from boundary effect. Second, to confirm that GATA acts as an enhancer blocker and not a repressive element, we performed RNA in situ hybridization against miniwhite , whose access to ftz is uninterrupted by GATA and found that ftz drove miniwhite to the same levels before and after flipping-out GE element ( Fig. 3b ). These results confirm the enhancer blocker activity associated with GATA SSR and rule out any repressive function associated with them. 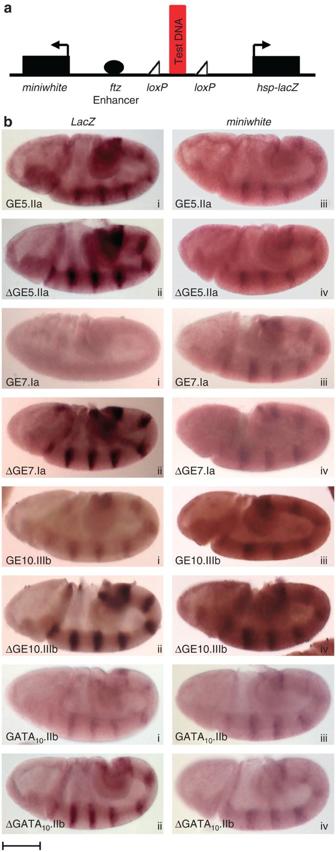Figure 3: GATA is an enhancer blocker and not a repressive element. (a) A schematic of the various elements on the transgene with respect to the reporterlacZ.(b) RNAin situhybridization forlacZandwhitegenes in the initial and flipped-out versions of corresponding lines. Left column shows that low levels of LacZ in the initial lines (i) are clearly enhanced when GE region is flipped out (ii). In the right column, however, white levels do not show enhanced expression in flipped-out lines (iv) when compared with initial lines (iii). The scale bar drawn on bottom left of the panel measures 100 μm in length. Figure 3: GATA is an enhancer blocker and not a repressive element. ( a ) A schematic of the various elements on the transgene with respect to the reporter lacZ. ( b ) RNA in situ hybridization for lacZ and white genes in the initial and flipped-out versions of corresponding lines. Left column shows that low levels of LacZ in the initial lines (i) are clearly enhanced when GE region is flipped out (ii). In the right column, however, white levels do not show enhanced expression in flipped-out lines (iv) when compared with initial lines (iii). The scale bar drawn on bottom left of the panel measures 100 μm in length. Full size image GE prevents genomic enhancer–promoter communication Among the various GE transgenic lines that we generated, one had the insertion at the optomotor blind ( omb ) locus (referred to as GE7.Ia or omb line) identified by the characteristic bipolar expression pattern of reporter miniwhite gene in the eyes ( Supplementary Fig. S4a ). Specific expression pattern of the omb gene is already known in the eye, wing and leg imaginal discs and their corresponding enhancers have also been mapped [26] . We sequenced this line using inverse PCR to map the precise insertion site of the transgene ( Fig. 4a ), thus enabling us to study whether GATA can prevent interaction between native enhancers and promoters. The optic lobe region (OLR) enhancer of omb that is downstream to lacZ , and, therefore, its access to hsp70-lacZ not interrupted by GE, drives the expression of lacZ reporter gene in, both, initial ( Fig. 4a ) and flipped-out lines ( Fig. 4a ). The slight reduction in the LacZ staining in the optic lobe of the flipped-out omb line can be reasoned as the titration of the OLR towards the omb and miniwhite genes as compared with the initial line, where OLR is dedicated only to the lacZ. On the contrary, the leg, eye and wing imaginal discs that show very little or no LacZ staining in the initial line ( Fig. 4b ), showed increased levels of lacZ expression upon flipping-out the GE ( Fig. 4c ). This implies that GE prevents these native omb enhancers from accessing the hsp70 promoter that drives lacZ . 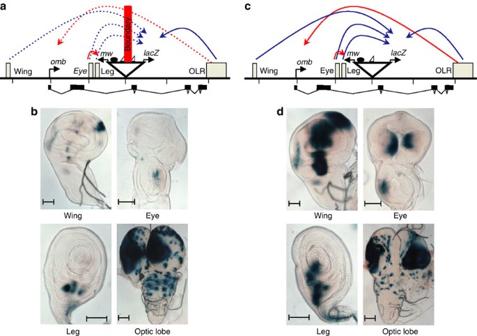Figure 4: GE prevents multiple enhancer–promoter communications in the native genomic context. Relative locations of the enhancers (wing, eye, leg and optic lobe regulatory region) of theombtranscription unit with respect to the reporter construct are shown (a). Dotted blue arrows show enhancer–promoter interactions interrupted by GE boundary while solid arrows show uninterrupted interactions. LacZ staining of wing, eye and leg imaginal discs showed no or minimal level oflacZexpression, indicating that the corresponding enhancers were blocked by the GE, while the OLR located at the other end of the insert was unaffected by GE, leading to high expression oflacZin optic lobes (b). In the flipped-out line, absence of GE allowed all enhancers to access thehsp70-lacZgene (c) as seen by the prominent expression oflacZgene in the corresponding discs (d). The scale bar drawn on bottom of the individual images measures 50 μm in length. Figure 4: GE prevents multiple enhancer–promoter communications in the native genomic context. Relative locations of the enhancers (wing, eye, leg and optic lobe regulatory region) of the omb transcription unit with respect to the reporter construct are shown ( a ). Dotted blue arrows show enhancer–promoter interactions interrupted by GE boundary while solid arrows show uninterrupted interactions. LacZ staining of wing, eye and leg imaginal discs showed no or minimal level of lacZ expression, indicating that the corresponding enhancers were blocked by the GE, while the OLR located at the other end of the insert was unaffected by GE, leading to high expression of lacZ in optic lobes ( b ). In the flipped-out line, absence of GE allowed all enhancers to access the hsp70-lacZ gene ( c ) as seen by the prominent expression of lacZ gene in the corresponding discs ( d ). The scale bar drawn on bottom of the individual images measures 50 μm in length. Full size image Further, we used the omb line as a tool to test whether GE can prevent enhancer–promoter interactions in their endogenous context also. We checked the expression of omb gene in the optic lobe by RNA in situ hybridization in the initial and flipped-out omb lines to see that omb gene expression decreases markedly when the access of OLR is blocked by GE. In the flipped-out line, OLR gets access to omb gene and thus an increase in the level of expression is seen ( Supplementary Fig. S4b ). On comparison of Fig. 4b and Supplementary Fig. S4b , it also becomes clear that GATA boundary function is independent of its orientation as in the former, we see that wing, eye and leg enhancers are unable to drive the lacZ expression while in the latter we see that the OLR enhancer, which is on the other side of the GE, is blocked from driving omb gene in the optic lobe. GATA does not act as heterochromatin–euchromatin barrier Chromatin domain boundaries are of two types—enhancer blockers and heterochromatin–euchromatin barriers. To test whether GATA SSR possessed the barrier activity also, we conducted the transgene protection assay in stable cell lines using NIH3T3 mouse fibroblast cell line and K562 human erytholeukaemia cell line with GATA 10 and GE7 as test fragments ( Supplementary Figs S5 and S6 ). The barrier assay we used is based on the fact that upon drug withdrawal, transgenes in the genome get silenced over a period of time by the gradual spread of nearby repressive/heterochromatic activity and that if the transgene is flanked by barrier elements that can block the spread of repressive activity, they can stay active for longer periods [27] . We found that although both GATA 10 and GE7 test fragment-containing transgenes were active to start with, none of them protected the reporter from getting silenced. GE7, however, showed a varying rate of silencing of the reporter gene in NIH3T3 cell line experiment, seen as high s.d. at early time points, which may indicate a weak barrier activity ( Supplementary Fig. S5b ). Even if it is so, this weak barrier activity is likely to be due to the non-GATA sequences of GE7, as GATA 10 did not show this activity. GATA failed to function as a barrier in K562 cell line also ( Supplementary Fig. S6a ). As these assays were done using a heterogeneous population of cells, we decided to confirm the lack of barrier activity using single-cell-derived lines of GATA 10 in K562. These clonal cell lines also failed to show any transgene protection as the reporter activity came down steadily after drug withdrawal ( Supplementary Fig. S6b ). From these results, we conclude that GATA SSR does not function as a barrier and that it only functions as an enhancer blocker boundary. Accumulation of the large proportion of repeats in complex eukaryotes, with SSRs reaching up to 3% in human genome [28] , but almost a similar number of genes may suggest that a lot of the complexity can be attributed to the recruitment of SSRs and other repeats as a tool in complex regulatory mechanisms. Presence of many SSR-binding proteins [29] , [30] , [31] further strengthens the view that these repeats may have functional relevance. One of the major SSRs in vertebrates, the GATA tetranucleotide, has many unique features such as preferred higher occurrence of (GATA) 10–12 , greater abundance on the mammalian Y chromosome and close association with developmentally regulated genes [9] , [10] . We here show that these GATA elements function as enhancer blocker elements that can demarcate functional domains in the genome. Our boundary assays show that GE could prevent enhancer–promoter interactions in human cell line and Drosophila melanogaster , indicating that the function of GATA is conserved and that the basic machinery involved in GATA function as a boundary is maintained in both invertebrates and vertebrates. By using synthetic GATA as the test element, we show that GATA repeats alone are sufficient for the boundary activity. Finally, using the omb line we show that GE can stop the interactions between enhancers and promoters in their native genomic context too. This suggests that the boundary activity of GATA is not a mere transgenic phenomenon but rather it reflects the functional significance of genomic GATA repeats as boundary elements. Our results also show that although GATA repeats block enhancer–promoter interactions, they fail to prevent the spread of heterochromatin into euchromatin making GATA SSR an exclusive enhancer blocker boundary element. A neutral boundary is not expected to affect expression of nearby genes unless located between the enhancer and the promoter driving that gene. In our experiments in human cells, we show that GATA represses reporter expression only when placed in between enhancer and promoter, and not when it is present upstream to the enhancer. In the fly system, we looked for both lacZ and miniwhite expression in the same stage by RNA in situ hybridization and found that only lacZ expression goes down as its interaction with the enhancer is interrupted by GE placed in between them while miniwhite expression remains unchanged. We conclude, therefore, that GATA is a neutral boundary and not a repressive element. We, in this study, show that GATA SSR can act as an enhancer blocker in multiple cell/tissue types, developmental stages and across species. Our results for the first time assign a direct role for SSRs in genome organization and formation of functional domains in complex organisms, and support the emerging view that repeats may not be ‘junk DNA’ and, instead, may constitute functionally relevant elements of the complex genomes. An obvious advantage that such repetitive functional elements may offer is that clustering of boundaries defined by repetitive elements, like the other known boundaries [32] , [33] , creates the possibility of bringing together large number of loci together in the nuclear compartment for coordinated expression and also provides a possible mechanism in which few factors can control coordinated expression of genes by choosing repeats as their targets [34] . As GATA repeats are also transcribed [35] , they may involve proteins that could utilize the transcripts made from them. Further, as repeats are more vulnerable to mutations and instability [36] , [37] , they can become a handy tool for the cell to bring about fine tuning of gene regulation and to give evolutionary pace to repeat-containing organisms. Further studies will be needed to explore these possibilities which may help us understand the evolution of complexity in the context of genomic organization and complex regulation of genes. DNA constructs The standard extraction protocol was followed for isolation of genomic DNA from human (male) blood sample, which included lysis, RNaseA and proteinaseK digestions, followed by phenol/chloroform extraction and precipitation. GEs from human Y chromosome were amplified using different GE primer pairs ( Supplementary Table S2 ) and cloned in PCR cloning vector InsT/A (Fermentas). Test fragments were cloned into the LML ( loxP-MCS-loxP ) vector in between the loxP sites. For the enhancer blocker assay in human cell line, the Xho I fragments from LML were cloned into the modified pJC54 vector whereas for the repressor assay the fragments were amplified and cloned into Nde I site upstream to the enhancer. For Drosophila transgenic constructs, Xho I fragments from LML were inserted at Xho I site of the ftzEN:hsp70/lacZ (pCfhL) vector [23] ( Fig. 2 ). Enhancer blocker and repressor assay in human cell line Enhancer blocking was tested using the colony formation assay in K562 cells [16] . For this assay, GE7, GE10, GE10MAR, GE10GATA and GATA 10 fragments were inserted between the mHS2 enhancer and the γ -globin promoter of the mHS2EN: γ g/neomycin vector for enhancer blocker assay and upstream to the mHS2 enhancer for the repressor assay. Equal amounts of DNA of each construct were electroporated into equal number of K562 cells, thus ensuring comparable transfection efficiencies. These transfected cells were then selected on neomycin for 2 weeks and plated to count the number of neomycin-resistant colonies. The experiment was done thrice to ensure reproducibility of the results. These results were averaged and ratios of number of colonies on neo + and neo − plates were plotted along with errors bars based on their s.e.m. Transgene protection assay Transgene protection or barrier assay construct consists of reporter green fluorescent protein (GFP) driven by CAGG promoter flanked by either GE7 or GATA 10 on both sides to be used as test fragments while the construct without any flanks was used as a negative control. The GEs were excised from Drosophila enhancer blocker vector, that is, pCfhL, and cloned in LMBP4800 vector modified to contain Not I and Xho I sites. Blasticidin gene was PCR amplified and cloned into a Sal I site downstream to the GFP and the subsequent GE of this barrier assay vector for selection of transfectants ( Supplementary Table S2 and Supplementary Fig. S2a ). NIH 3T3 cells and K562 cells were transfected using Lipofectamine 2000 (Invitrogen) according to the manufacturer’s protocol. Stable transfectants were selected using 17 μg ml −1 blasticidin drug for NIH3T3 and 25 μg ml −1 for K562 for 2 weeks, after which the drug was withdrawn to follow the time course of disappearance of GFP. Single cell clones in K562 cell line were also isolated for the same. The cells were monitored for GFP for 40 days post drug withdrawal and the GFP was measured periodically by fluorescence-activated cell sorting analysis using MoFlo (Dako Cytomation). The per cent GFP was normalized to day 0 readings and were plotted as shown in Supplementary Figs S5b and S6 . Gel shift assay Radiolabelled DNA (about 1 fmol) was incubated with nuclear extract for 30 min (15 min on ice and 15 min at room temperature) 1 × binding buffer (25 mM HEPES (pH 7.6), 100 mM NaCl, 1 mM DTT, 0.1 mM PMSF and 10% glycerol), 10 μg yeast tRNA, 0.5 μg polydIdC and 0. 5 μg Escherichia coli sonicated genomic DNA. Specific cold competitor was added wherever mentioned. The DNA–protein complexes were resolved using 5% polyacrylamide gel (39:1 acrylamide: bis-acrylamide). Enhancer blocker assay in Drosophila Transgenic lines were generated, following the standard protocol [38] , [39] . All the pCfhL constructs having GE DNA were injected (0.5 mg ml −1 ) into embryos of Drosophila carrying transposase ( w − y − Δ 2 – 3kstb ). The test element was flipped out by crossing the flies bearing the transgene with the strain expressing Cre recombinase (Bloomington stock no. 766) (ref. 40 ). Inverse PCR was performed following the published protocol [41] to determine the precise insertion site for useful lines. Embryos (0–12 h) were collected and stained for β-galactosidase ( lacZ ) activity according to the protocol [42] with minor changes [43] as outlined. Briefly, 0- to 12-h-old embryos were dechorionated in 50% bleach (sodium hypochlorite), washed and fixed in heptane saturated with 25% glutaraldehyde for 20 min. The fixed embryos were washed with PBSTx (PBS+0.3% Triton X 100) thoroughly followed by a single wash with pre-warmed X-gal staining buffer (7.2 mM Na 2 HPO 4 , 2.8 mM NaH 2 PO 4 , 150 mM NaCl, 1 mM MgCl 2 , 3 mM K 3 [Fe(CN) 6 ], 3 mM K 4 [Fe(CN) 6 ]). The embryos were then incubated in staining buffer containing 1% X-gal (Sigma) till good staining pattern develops (2–10 h). Imaginal discs were fixed in 4% paraformaldehyde for 20 min at room temperature, washed twice in PBSTx and processed for LacZ staining as described for embryos. All the LacZ activity-stained embryos were imaged with Leica Stereomicroscope. RNA in situ hybridization To see the expression pattern of miniwhite , lacZ and omb in the embryos and/or discs, in situ hybridization was carried out using messenger RNA-specific RNA probes. The desired regions were PCR amplified using the primer pairs ( Supplementary Table S2 ), cloned into pGEMT Eazyvector (Promega), digUTP-labelled RNA probes were made using Roche in vitro transcription kit and used for in situ hybridization [44] . Proteinase K treatment instead of acetone treatment was adopted for the discs [45] . The probes were detected using alkaline phosphatase-conjugated anti-dig antibody as described in the Roche DIG application manual for in situ hybridization. All RNA in situ hybridized embryos were imaged using Zeiss Axioplan microscope. How to cite this article: Kumar, R. P. et al. GATA simple sequence repeats function as enhancer blocker boundaries. Nat. Commun. 4:1844 doi: 10.1038/ncomms2872 (2013).